Ionophore constructed from non-covalent assembly of a G-quadruplex and liponucleoside transports K+-ion across biological membranes 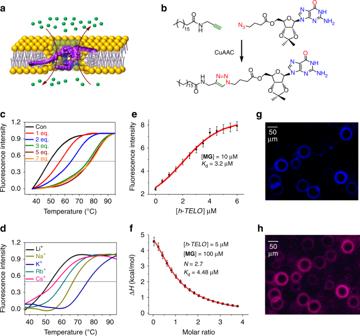Fig. 1: Interaction ofMGwithh-TELO. aScheme showing K+transport by theh-TELOionophore within a lipid membrane. Theh-TELOG-quadruplex is anchored to the lipid membrane by guanosine derivatives (MG) containing lipophilic chains (purple). The K+-ions are depicted as green balls and Cl−-ions are shown as orange balls.bScheme outlining the synthesis of monoguanosine derivative (MG).cMelting profile ofh-TELOstabilized by increasing concentration (0–7 equiv.) ofMGin 10 mM HEPES, 100 mM KCl buffer, pH 7.4 (Tmofh-TELOis 49 °C in the same buffer).dMelting profile of 3:1MG/h-TELOin the presence of different metal ion containing buffer (10 mM HEPES, pH 7.4, containing 100 mM LiCl, NaCl, KCl, RbCl, and CsCl, respectively).eFluorescence intensity profile ofMGupon titration with increasing concentration ofh-TELOin 10 mM HEPES, 100 mM KCl buffer, pH 7.4.fITC titration ofMGwithh-TELOin 10 mM HEPES, 100 mM KCl buffer, pH 7.4. Fluorescent images (λem= 355 nm) of lipid vesicles (GUV)gwithMG/h-TELOandhco-staining withMG/h-TELOand membrane-binding dye, Nile red. Source data are provided as a Source Data file. Data are means ± SD (n= 3). The selective transport of ions across cell membranes, controlled by membrane proteins, is critical for a living organism. DNA-based systems have emerged as promising artificial ion transporters. However, the development of stable and selective artificial ion transporters remains a formidable task. We herein delineate the construction of an artificial ionophore using a telomeric DNA G-quadruplex ( h-TELO ) and a lipophilic guanosine ( MG ). MG stabilizes h-TELO by non-covalent interactions and, along with the lipophilic side chain, promotes the insertion of h-TELO within the hydrophobic lipid membrane. Fluorescence assays, electrophysiology measurements and molecular dynamics simulations reveal that MG / h-TELO preferentially transports K + -ions in a stimuli-responsive manner. The preferential K + -ion transport is presumably due to conformational changes of the ionophore in response to different ions. Moreover, the ionophore transports K + -ions across CHO and K-562 cell membranes. This study may serve as a design principle to generate selective DNA-based artificial transporters for therapeutic applications. The transport of ions across the semi-permeable cell membrane is a fundamental biological process that play key roles in signal transduction, nerve impulse, muscle contraction, hormonal regulation, and apoptosis [1] , [2] . Dysfunctional ion transport activity may cause Alzheimer's disease, Parkinson's disease, cystic fibrosis, vision disorders etc. [3] . The naturally occurring ion channels selectively transport a particular type of metal ions across the cellular membrane. To mimic the function of these protein-based ion channels, artificial ionophores are being developed. Several synthetic scaffolds [4] , [5] , [6] , [7] , [8] , [9] , [10] , [11] , [12] , [13] , polypeptides [14] , nanopores [15] , [16] , and even DNA-based materials [17] , [18] , [19] , [20] have been reported [21] , [22] , [23] , [24] , [25] , [26] . Specifically, the idea of using DNA to imitate the activity of membrane-protein functions has generated wide attention due to their enhanced ability to form predetermined structures with predictable mechanical properties [27] , [28] , [29] , [30] . Membrane-spanning DNA ionophores of different dimensions have been constructed using a single duplex DNA [31] or programmed assembly of multiple duplex DNA sequences [32] . These DNA-based ionophores can mediate efficient ion transport and hence they are crucial to understand the biological role of their natural counterparts [33] . In addition, ionophores find important applications in a wide range of therapeutics (antibiotics, antimicrobials etc.) [34] , [35] , DNA sequencing, sensors [36] , [37] , and delivery systems [38] . Unlike natural ion channels, artificial ionophores show low selectivity and lack stimuli-responsive behavior. Therefore, developing artificial ionophores with preference for a particular ion is an attractive area of research [39] , [40] , [41] , [42] . In this backdrop, cation-rich four stranded G-quadruplex DNA [43] presents an ideal scaffold to construct cation-selective ionophores. The basic structural unit of a G-quadruplex is G-quartet, made of four guanines associated by Hoogsteen type of hydrogen bonding. The G-quartets stack upon each other to form G-quadruplex, which is further stabilized by metal ions (e.g., K + , Na + etc.). Synthetic guanosine derivatives that can self-assemble to form columnar assemblies of G-quartets have been reported to transport cations across lipid bilayers [44] , [45] , [46] , [47] , [48] . In contrast to synthetic guanosine derivatives, the exterior of a G-quadruplex DNA contains negatively charged phosphate backbone. As a result, the insertion of a charged G-quadruplex structure in the hydrophobic lipid membrane is energetically unfavorable. We hypothesized to use non-covalent assembly of a G-quadruplex with a lipophilic ligand to construct artificial ionophores. This method excludes the rigorous development of covalently linked lipophilic DNA molecules for the insertion into the membrane. In our approach, an endogenous human telomeric G-quadruplex DNA ( h-TELO ; PDB: 1KF1) [49] is inserted into the lipid membrane by a synthetic guanosine-derivative MG containing a lipophilic side chain (Fig. 1a ) [50] , [51] . The potential of MG / h-TELO ionophore to transport K + in a stimuli-responsive manner is validated using fluorescence-based vesicle assay, voltage–clamp conductance measurements, and MD simulations. Finally, we shed light on ion transport across the cell membrane and the probable mechanism of ion transport under external conditions. Fig. 1: Interaction of MG with h-TELO . a Scheme showing K + transport by the h-TELO ionophore within a lipid membrane. The h-TELO G-quadruplex is anchored to the lipid membrane by guanosine derivatives ( MG ) containing lipophilic chains (purple). The K + -ions are depicted as green balls and Cl − -ions are shown as orange balls. b Scheme outlining the synthesis of monoguanosine derivative ( MG ). c Melting profile of h-TELO stabilized by increasing concentration (0–7 equiv.) of MG in 10 mM HEPES, 100 mM KCl buffer, pH 7.4 (T m of h-TELO is 49 °C in the same buffer). d Melting profile of 3:1 MG/ h-TELO in the presence of different metal ion containing buffer (10 mM HEPES, pH 7.4, containing 100 mM LiCl, NaCl, KCl, RbCl, and CsCl, respectively). e Fluorescence intensity profile of MG upon titration with increasing concentration of h-TELO in 10 mM HEPES, 100 mM KCl buffer, pH 7.4. f ITC titration of MG with h-TELO in 10 mM HEPES, 100 mM KCl buffer, pH 7.4. Fluorescent images ( λ em = 355 nm) of lipid vesicles (GUV) g with MG/ h-TELO and h co-staining with MG/ h-TELO and membrane-binding dye, Nile red. Source data are provided as a Source Data file. Data are means ± SD ( n = 3). Full size image Synthesis of lipophilic guanosine MG The lipoguanosine MG containing a 17-carbon long lipophilic side chain was synthesized using Cu(I)-catalyzed azide−alkyne 1,3-dipolar cycloaddition of an azido functionalized guanosine and an alkyne functionalized stearic acid. The reaction was carried out using Na-ascorbate and CuSO 4 ·5H 2 O in t -BuOH/H 2 O (1:1) to obtain the triazole-linked lipophilic guanosine derivative MG in 52% yield (Fig. 1b ; Supplementary Fig. 1 ). Binding studies of MG with h-TELO G-quadruplex First, we investigated the interaction of MG with h-TELO G-quadruplex using melting analysis by Förster resonance energy transfer (FRET) [52] , fluorometric titrations, and Isothermal calorimetry (ITC). We used a 22-mer h-TELO sequence that folds into a G-quadruplex in K + -buffer (PDB ID: 1KF1). FRET-based melting profiles of the dual-labeled (FAM and TAMRA at 5′- and 3′-ends, respectively) h-TELO G-quadruplex were monitored in the presence of incremental concentrations of MG (0–7 equiv.). Upon addition of MG , h-TELO showed an increase in melting temperature ( T m ) with saturating Δ T m values (Δ T m = 27 °C; T m = 76 °C) at 3 equiv. ligand concentrations, suggesting that MG could considerably stabilize h-TELO G-quadruplex (10 mM HEPES, 100 mM KCl, pH 7.4) (Fig. 1c ). The melting analysis of MG/ h-TELO in the presence of different alkali metal cations (Li + , Na + , K + , Rb + , and Cs + ) revealed that MG/ h-TELO exhibited the highest T m value in K + -ions ( T m = 76 °C) compared to other ions ( \({T}_{\mathrm{m}}^{{\mathrm{Na}}}\) = 67 °C; \({T}_{\mathrm{m}}^{{\mathrm{Li}}}\) = 52 °C; \({T}_{\mathrm{m}}^{{\mathrm{Cs}}}\) = 55 °C; \({T}_{\mathrm{m}}^{{\mathrm{Rb}}}\) = 59 °C) at 3 equiv. ligand concentration (Fig. 1d ). Next, fluorescence studies revealed that MG is weakly fluorescent. When MG (10 μM) ( λ ex = 265 nm) was titrated with h-TELO (0–6 μM) in 100 mM KCl, 10 mM HEPES at pH 7.4, a dose-dependent increase in fluorescence intensity ( λ em = 355 nm) of MG was observed (Fig. 1e ; Supplementary Figs. 2 , 3 ). The dissociation constant ( K d ) was calculated to be 3.2 μM. The Job’s plot analysis revealed that MG binds to h-TELO with a 3:1 stoichiometry (Supplementary Fig. 4 ). The ITC data further suggested a 3:1 binding stoichiometry between MG and h-TELO ( K d = 4.48 μM) (Fig. 1f ; Supplementary Fig. 5 ). Membrane localization of MG/ h-TELO As MG showed “turn-on” fluorescence upon binding to h-TELO , we employed fluorescent imaging to examine the localization of MG / h-TELO in giant unilamellar vesicles (GUV, lipid bilayer). GUVs were prepared using a 9:1 mixture of lipid and cholesterol. Upon addition of 20 μM MG/ h-TELO , blue rings were observed around the GUVs. Interestingly, these blue rings were co-localized with the membrane staining dye Nile red, indicating that MG / h-TELO is inserted in the membrane (Fig. 1g, h ). However, no fluorescence was observed when GUVs were treated with either h-TELO or MG . Thus, the insertion of MG / h-TELO within lipid bilayer could be detected without using fluorescent labels. Ion-transport activity of MG/ h-TELO by fluorescence assay To evaluate the transport of alkali cations across the lipid bilayer, a fluorescence-based assay was performed using 8-hydroxypyrene-1,3,6-trisulfonic acid (HPTS) dye [53] (Fig. 2 ). Liposomes (large unilamellar vesicles (LUV), 100 nm diameter) were filled with a pH-sensitive dye HPTS ( λ ex = 460 nm, λ em = 510 nm) in 100 mM NaCl and HEPES buffer solution (10 mM, pH 6.4). The liposomes were then suspended in an external HEPES buffer solution (10 mM, pH 6.4) containing 100 mM KCl. A pH gradient, ΔpH = 1 (internal pH, pH in = 6.4; outside pH, pH out = 7.4) across the lipid bilayer was applied by the addition of NaOH. The formation of an ionophore by MG / h-TELO assembly was expected to induce a pH gradient collapse via H + efflux leading to an increase in the pH in of the vesicles. This efflux of H + ions triggers an influx of external cation (K + , Na + etc.) to maintain the equilibrium of electrical charge across the lipid bilayer. Complete destruction of the pH gradient was achieved by addition of 10% Triton X-100. The change in pH in of the vesicles was monitored by the change in the fluorescence of HPTS, which indicates cation transport across the lipid bilayer. The relative pH change was quantified upon addition of MG / h-TELO in the presence and absence of external pH gradient and subsequently the rate constants were calculated as described in Supplementary Information (Supplementary Fig. 6 ). Fig. 2: Fluorescence-based ion-transport assay. Change in normalized pH inside LUV (pH in ) as a function of time with increasing addition of MG / h-TELO (0–60 μM) in the presence of different metal ions and pH gradient. a Buffer composition, external: 10 mM HEPES, 100 mM KCl, pH 7.4; internal: 10 mM HEPES, 100 mM NaCl, pH 6.4. b Buffer composition, external: 10 mM HEPES, 100 mM NaCl, pH 7.4; internal: 10 mM HEPES, 100 mM KCl, pH 6.4. Change in normalized pH inside LUV as a function of time in the presence of MG / h-TELO (60 μM) using different external metal ions. c Buffer composition, external: 10 mM HEPES, 100 mM MCl (M = Na + , Li + , Cs + , NH 4 + , and K + ), pH 7.4; internal: 10 mM HEPES, 100 mM NaCl, pH 6.4. d Buffer composition, external: 10 mM HEPES, 100 mM MCl (M = Na + , Li + , Cs + , NH4 + , and K + ), pH 7.4; internal: 10 mM HEPES, 100 mM KCl, pH 6.4. e Pseudo-first-order initial constant rate as a function of final concentration of MG / h-TELO in the bilayer membrane. f Fractional activity Y = f([ MG / h-TELO ]) plotted for Na + and K + ions and the curves are the best fit from the Hill equation. Source data are provided as a Source Data file. Data are means ± SD ( n = 3). Full size image For each batch of experiments, a blank experiment in the absence of additives demonstrated that a basal level change in pH in was observed due to simple diffusion through the liposome bilayer. To exclude the possibility of vesicle rupture or fusion as a probable cause of change in pH in values, dynamic light-scattering studies were carried out at different time points. The uniformity of vesicle size at all time points confirmed that no fusion or rupture of vesicles took place upon addition of MG / h-TELO (Supplementary Fig. 7 ). Additional control experiments further revealed that there were insignificant changes in pH in either with free MG or h-TELO (Supplementary Fig. 8 ). The addition of MG/ h-TELO (60 μM) generated a rapid increase in pH in , indicating a fast efflux of proton and a high-influx rate for the external K + -ions (external buffer: 10 mM HEPES, 100 mM KCl, pH 7.4) (Fig. 2a ). However, when the external and internal buffers were reversed maintaining the pH gradient (pH in 6.4 and pH out 7.4), significantly slow change in internal pH was observed (Fig. 2b ). To investigate whether the change in pH in is dependent on concentration of MG/ h-TELO , we performed concentration-dependent HPTS assay. Upon incremental addition of MG/ h-TELO (0–60 μM), a dose-dependent increase in pH in (external buffer: 10 mM HEPES, 100 mM KCl, pH 7.4; internal buffer: 10 mM HEPES, 100 mM NaCl, pH 6.4) was observed which attained saturation at 50 μM concentration (Fig. 2a ). In contrast, MG/ h-TELO (60 μM) showed significantly lower activity when external KCl was replaced with NaCl (internal buffer: 10 mM HEPES, 100 mM KCl, pH 6.4) (Fig. 2b ). Using other alkali metal chlorides (LiCl and CsCl) and ammonium ions (NH 4 + ) in external buffer, minimal changes in internal pH were observed (Fig. 2c ). In addition, lucigenin assay suggested that MG/ h-TELO could not transport Cl − -ions (Supplementary Fig. 9 ). Furthermore, when 100 mM KCl was present in internal solution, a small change in internal pH, irrespective of different metal ions in external buffer was observed (Fig. 2d ). These experiments suggest that ionophores formed by MG/ h-TELO are responsive to K + -ions. The transportation activity for Na + and K + was then investigated by varying the concentration of MG/ h-TELO from 0 to 60 μM. MG/ h-TELO exhibited pseudo-first-order kinetics for the transport of both cations (Supplementary Figs. 10 , 11 ). Rate constant ( k obs ) values were plotted against increasing concentrations of MG/ h-TELO (Fig. 2e ). The transport rates for K + ( k K + ) were found to be saturated at 50 μM MG/ h-TELO concentration, whereas no saturation in transport rates for Na + -ions ( k Na + ) was obtained. At this concentration (50 μM), a ~10-fold higher transport rate for K + -ions ( k K + = 0.062 s −1 ) was observed over Na + ( k Na + is 0.0062 s −1 ). To determine the effective concentration of MG/ h-TELO required to obtain 50% of transport activity (EC 50 ) and the stoichiometry of the transport process (Hill coefficient), the fractional activity at 300 s for each concentration was plotted against the concentration of MG/ h-TELO (Fig. 2f ). Hill analysis of the plots revealed that the EC 50 values for K + and Na + were 19 μM and 54 μM, respectively. The Hill coefficients ( n ) for both cations were also found to be different: 1.76 for K + and 0.81 for Na + . Together, these results indicate that ionophores formed by MG / h-TELO preferentially transport K + -ions over other alkali metal ions. Next, the ability of MG/ h-TELO to transport cations in the absence of pH gradient (passive transport) was investigated using HPTS assay (Supplementary Figs. 12 , 13 ). Interestingly, this passive transport was activated only in the presence of cation concentration gradient across the lipid bilayer. In the presence of same internal and external buffer (containing 100 mM NaCl, pH 6.4), a negligible change in the internal pH was observed upon treatment with MG/ h-TELO (60 μM) ( t = 50 s), indicating no passive transport. However, when KCl was present in external buffer, passive transport was observed in a dose-dependent manner by addition of MG/ h-TELO (60 μM) ( t = 50 s). Interestingly, when KCl was present inside the vesicle (NaCl outside), passive transport was reversed. These results suggest that passive ion transport is dependent on the concentration gradient of K + -ions. In addition, safranin assay suggested that the passive ion transport by h-TELO ionophore can alter the transmembrane potential (Supplementary Fig. 14 ). Atomistic insight into the formation of MG/ h-TELO ionophore Equilibrium simulations were then performed to gain atomistic insights into the formation of ionophore in the membrane (Fig. 3 ). Simulations were performed by using parmbsc1 force field [54] implemented in GROMACS simulation packages [55] , [56] . The details of the simulation methodologies and validations of the force field for G-quadruplex and membrane simulations have been provided in the Supplementary Information (Supplementary Figs. 15 , 16 ). Equilibrium simulations of MG / h-TELO with different stoichiometries (1:1, 2:1, & 3:1) revealed that native G-quadruplex shows the highest stabilization in the presence of three molecules of docked MG , characterized by low root-mean-square deviation from the crystal structure throughout the simulation trajectory (Supplementary Fig. 17 ). This result complements FRET-based melting and isothermal calorimetry studies. During equilibrium simulation of MG/ h-TELO with a 3:1 stoichiometry, guanosine moieties of MG stack on the terminal quartet of G-quadruplex, while the long alkyl tails wrap the quadruplex along the groove region to form a highly stable assembly (Supplementary Fig. 18 ). MG/ h-TELO was then inserted within the membrane such that the K + -filled pore of the h-TELO was aligned along the Z -axis. The structure of the initial assembly is shown in Fig. 3a . During membrane insertion simulation, water molecules from the bulk came toward the h-TELO and hydrated the quadruplex structure within the lipid membrane. The MG/ h-TELO subsequently underwent large conformational transition to form highly stable ionophore. Once, water-filled pore was formed inside the membrane, the lipophilic chains of MG in the h-TELO were incorporated into the hydrophobic region of the lipid bilayer constituted by the fatty acid tails of phospholipid. Interestingly, among the three bound MG molecules, two of them anchor the h-TELO with the membrane, the third one wraps the DNA along the groove and its guanosine moiety perfectly stacks with the G-quartet providing additional stability to the G-quadruplex inside the pore. The charged phosphate backbone of the G-quadruplex was thus exposed within the membrane, which attract more and more water molecules from the bulk to solvate the G-quadruplex to form a water-filled channel within the membrane. Adjacent phospholipids also underwent structural rearrangements such that their phosphate head groups could face toward the water pore. This assembly was found to be highly stable throughout simulation. The formation of such water channel along the simulation trajectory is shown in Fig. 3a . Upper view of the supramolecular ionophore is shown in Fig. 3b . MG molecules played crucial role in stabilizing the h-TELO , apart from anchoring it within the membrane matrix. The guanosine moiety stabilized the G-quartet through stacking interactions (Fig. 3c ), and other polar groups of MG could form ~6–8 hydrogen bonds with the h-TELO (Fig. 3d ). In a control simulation using only h-TELO , it was observed that in the absence of MG , h-TELO diffused away from the water pore (Supplementary Fig. 19 ). Interestingly, the translational diffusion of the h-TELO increased in the absence of MG and it could not retain the G-quadruplex structure in the membrane. The stacking of G-quartets in the G-quadruplex was observed to be lost during the simulation timescale (Supplementary Figs. 19, 20 ). Fig. 3: MG/ h-TELO ionophore formation within lipid bilayer. a Process of pore formation around h-TELO within the lipid membrane. Initially, ligand-bound quadruplex (blue vdW representation) is placed within the lipid bilayer (gray stick) in a water box (red surface). b Final structure of the supramolecular quadruplex-based ion pore. Lipid bilayer is colored in green surface, whereas the water pore surrounding the quadruplex is shown in pink surface. h-TELO is shown in blue cartoon, and bound MG is shown in orange sticks. c Structure of MG/ h-TELO is shown. G-quadruplex is shown in cartoon representation, whereas bound ligand is shown in stick mode. d The number of hydrogen bonds between h-TELO and MG during the simulation of the ionophore is shown. e A representative snapshot of K + (blue) and Cl − (red) ion distributions in the simulation box is shown. Lipid bilayer is shown as gray transparent surface. f Density profiles of K + (blue) and Cl - (red) ions averaged over the entire 200 ns simulation trajectory are shown. g Potential of mean force profile for K + (blue) and Cl − (red) translocation across the simulation box ( Z -axis). Source data are provided as a Source Data file. Data are means ± SD ( n = 3). Full size image From equilibrium simulation, we further monitored the distribution of K + and Cl − ions by inserting MG / h-TELO in the lipid membrane in 200 mM KCl solution. A representative snapshot of K + (blue) and Cl − (red) ion distribution in the simulation box is shown in Fig. 3e , and the corresponding density profiles of the two ions averaged over the entire 200 ns simulation trajectory are shown in Fig. 3f . As evident from the figure, K + -ions were preferentially distributed around the phosphate groups of the bilayer. In addition, there was significant K + -ion density within the water pore. The peak in the K + -ion density profile within the water pore corresponded to its preferential distribution along the phosphate backbone of the G-quadruplex. In contrast, Cl − was distributed mostly in the bulk with no noticeable density within the water pore due to electrostatic repulsion from the negatively charged phosphate backbone of h-TELO . The potential of mean force calculation revealed that the free-energy of K + -ion movement from the bulk to the water pore was within the diffusion control limit, whereas free-energy barrier for the same translocation of a Cl − -ion was ~10 times higher (Fig. 3g ). Voltage-dependent ion-transport induced by the MG/ h-TELO To investigate voltage-dependent K + -ion transport activities of MG/ h-TELO across the lipid membrane; ionic current recording studies were conducted as follows: phospholipid bilayers with 1 M KCl containing buffer at the cis and trans chambers were prepared, and the current was recorded after addition of MG/ h-TELO (60 μM) to the cis chamber. Interestingly, we observed transient fluctuations between distinct current values. From the histogram, it is clear that the current fluctuation corresponds to two states of the ionophore: a fixed closed state (mostly around 0 pA) and variable open states depending upon the sign and magnitude of the holding potential (Fig. 4a, b ). The conductance values are calculated to be 1.6 ± 0.4 nS in the presence of 10 mM HEPES buffer containing 1 M KCl (pH 7.4). In addition, MG/ h-TELO exhibited significantly high transport activity with long opening periods at +80 mV holding potential (Supplementary Fig. 21 ). However, no fluctuation in current was observed in control experiments using  either MG or h-TELO (Supplementary Fig. 22 ). When KCl was replaced with NaCl in the buffer, MG / h-TELO exhibited considerably weaker transport activity (Supplementary Fig. 21 ). Other chlorides like LiCl, RbCl, CsCl, and NH 4 Cl showed negligible transport activity (Supplementary Fig. 23 ). Fig. 4: Ion conductance studies across the lipid bilayer by MG/ h-TELO . Single-channel current traces recorded at +20 mV ( a ) and −50 mV ( b ) holding potentials in 1 M symmetrical KCl solution in the presence of MG/ h-TELO (60 μM). All point histograms generated from the corresponding current traces at +20 mV and −50 mV have been presented on the right. c I − V plot using a voltage ramp (−60 mV to +60 mV) in 1 M symmetrical KCl solution (black line) in the presence of MG/ h-TELO (60 μM). Data are means ± SD ( n = 3). d Cumulative currents through the transmembrane pore resulting from the application of external electric fields. Orange, maroon, pink, black, light blue, deep blue, green, and purple color represent +100 mV, +75 mV, +50 mV, +25 mV, −25 mV, −50 mV, −75 mV, and −100 mV applied voltage biases. e Cumulative current flow for K + ions under the applied voltage biases of +100 mV (green), −100 mV (purple) and for Cl − ions under the applied voltage biases of +100 mV (black), −100 mV (pink). f Current/voltage characteristics of supramolecular transmembrane ionophore computed from molecular dynamics simulations under different applied voltage biases. Source data are provided as a Source Data file. Data represented as Mean ± SD ( n = 4). Full size image In order to understand the K + -ion transport property, a current−voltage relationship ( I − V plot) was further derived (Fig. 4c ). The I − V plot follows an ohmic relation with symmetrical currents at negative and positive polarity ranging from −50 mV to +50 mV. The linear fit of the plot showed a slope value of 1.4 nS. Atomistic insight into the ion-transport by MG/ h-TELO Ion conductance simulations were next carried out to provide atomistic insight into the ion transport across the lipid bilayer through the ionophore formed by MG / h-TELO . NPzAT simulations were carried out in 200 mM KCl solution, in line with fluorescence-based ion-transport assay, to measure current flow in the presence of an external electric field along the Z -axis. The system was simulated at +100, +75, +50, +25, −25, −50, −75, and −100 mV transmembrane biases for ∼ 80 ns at each bias. During initial simulation phases, ions and water molecules in the bulk rapidly reoriented under the influence of an external electric field and attained stationary phase, where the applied electric field essentially generated transmembrane voltage bias. Therefore, initial 30 ns of simulation trajectories were not considered during cumulative current calculations to ensure that all the systems attain stationary state. Cumulative current was conducted by a method originally introduced by Aksimentiev et al. [57] , and later classified as total intensity method by Faraudo et al. [58] . Evident from Fig. 4d , the cumulative total current flow linearly increased with simulation time under the effect of applied voltage which implicate that all the system attained stationary state. We then calculated the contribution of K + and Cl − on total current flux. In all applied voltage bias, the current conducted through the system was contributed from the K + -ion translocations only. Current conducted by the Cl − ion was negligible in all applied voltage bias indicated its movement was primarily diffusion controlled and unaffected by the transmembrane voltage bias (Fig. 4e ). Therefore, Cl − could not penetrate the transmembrane pore, in line with equilibrium simulation and experiments. Calculated I−V plot (Fig. 4f ) from the simulation within +100 mV to – 100 mV region was found to be linear thus follow ohmic relation. The average conductance calculated from the simulation was 1.075 nS, which is in excellent agreement with the conductance obtained from voltage–clamp experiments. Proposed mechanism for ion transport by the MG/ h-TELO The plausible mechanism for the cation transport (K + ) in lipid vesicles by MG / h-TELO with pH gradient is interpreted based on the experimental data (Fig. 5 ). Initially, Na + ions filled vesicles are placed in K + -ion buffer to create an ion gradient across the lipid bilayer. The addition of MG / h-TELO induces rapid reorientation of phosphate head groups in the bilayer to form ionophores (Fig. 5a ). A pH gradient across the lipid membrane of the vesicles (pH in = 6.4 and pH out = 7.4) is induced by adding NaOH in the medium. This triggers a H + efflux, followed by a K + influx down the concentration gradient (to maintain the charge equality) showing hyperbolic increase in pH in values with time (Fig. 5b ). The plateau region is reached due to a slow H + /K + exchange that equillibrates the K + -ion concentration and pH inside the vesicle (small amounts of Na + efflux may also take place down the concentration gradient). Importantly, when MG was heat annealed in K + solution and added to the vesicles, no significant ion transport was observed. This is in accordance with CD studies which show that MG has a very low efficiency to form G-quadruplex like structures compared with diguanosine derivatives [44] reported before (Supplementary Fig. 24 ). The addition of Triton X solubilizes lipid membranes to finally equilibrate the ionic concentration and pH in the entire solution. In the presence of Na + in external buffer, small changes in pH in values suggest that lower influx of Na + possibly retards H + efflux. In addition, the presence of other alkali cations (Li + , NH 4 + , and Cs + ) in external buffer shows negligible changes in pH in values, suggesting their reduced influx. In passive diffusion experiments (K + outside and Na + inside), MG / h-TELO activates K + influx down the concentration gradient along with a H + efflux, and membrane polarization takes place (observed from Safranin O assay) as sharp increase in pH in values are observed (Fig. 5c ). When the internal and external buffer is exchanged (K + inside and Na + outside), a fast K + efflux followed by a H + influx takes place as evidenced by a sharp decrease in pH in values. However, the changes in pH in values are much higher by applying external pH gradient. Fig. 5: Proposed mechanism for ion transport in fluorescence assay. Schematic representation showing a the formation of water-filled ionophore in the lipid bilayer by rearrangement of lipid molecules upon insertion of MG / h-TELO . The lipophilic chains of MG anchors the MG / h-TELO to stabilize the ionophore. b The stepwise ion transport (left to right) by pH-dependent transport (top) and; c passive diffusion (bottom). Full size image The nature of ion transport by MG / h-TELO has been elucidated by HPTS, Lucigenin, Voltage clamp and MD simulation studies. The MD simulation studies along with the negative Lucigenin assay data strongly suggest that the conducting ions are cationic metal ions and not anionic Cl − ions. This may be due to the presence of negatively charged phosphate backbone of G-quadruplex which repels the anions from entering the water-filled channel. MG/ h-TELO as K + ionophore To decipher the origin of the high transport rates of MG / h-TELO ionophore for K + ions, we examined three systems: K + -stabilized MG / h-TELO in KCl and NaCl media, respectively, and Na + -stabilized MG / h-TELO in NaCl media.The systems were simulated using same protocol with the applied external electric field of +75 mV and −75 mV and ion-conductance values were calculated. These studies indicate that the K + -stabilized MG / h-TELO ionophore exhibits higher flow of cumulative current for KCl over NaCl solution. In KCl solution, the cumulative total current flow linearly increases with simulation time under the effect of applied voltage in either direction, implicating the system attained stationary state and there is steady flow of current (Fig. 6a ). The K + -stabilized MG / h-TELO may transport different monovalent ions, depending on the mobility of the ions. However, for Na + -stabilized MG / h-TELO , steady flow of current is not observed, and stationary state is not attained. Fig. 6: MG/ h-TELO as K + ionophore. Molecular dynamics simulations of MG / h-TELO in KCl and NaCl electrolyte solutions, represented by purple and orange color, respectively. The Na + -stabilized MG / h-TELO in NaCl electrolyte solution is represented by green color. a Cumulative current flow computed for the three systems under the applied voltage biases of +75 mV, rendered in the dark color and −75 mV, represented in light color. b 2-D scatter plot of root-mean-square deviation (RMSD) and radius of gyration (R g ) obtained from the equilibrium simulations. Variations of the distance vector along the Z -axis between tetrads 1 & 2 c and tetrads 2 & 3 d are shown for MG / h-TELO ionophore embedded in the lipid bilayer in three different conditions obtained from the simulations. e I–V curves generated from the tail currents of the traces in different buffer conditions. Bi-ionic conditions were used: 10 mM HEPES buffer containing 0.150 M KCl in the cis side and 0.150 M different metal chlorides (LiCl, NaCl, KCl, RbCl, and CsCl) in the trans side. f Permeability ratios of MG / h-TELO obtained for different monovalent cations with respect to K + ion. Source data are provided as a Source Data file. Data represented as mean ± SD ( n = 4). Full size image Next, the structure of the MG / h-TELO ionophore in these systems was assessed from the equilibrium simulations. These results show that MG / h-TELO ionophore exists in different conformations in response to K + and Na + ions. As evident from the 2-D RMSD-R g plot, an increase in RMSD and subsequent deviation of R g are observed in Na + -stabilized MG / h-TELO , suggesting perturbation of the native structure with simulation time (Fig. 6b ). We further quantified how different ions perturb the G-quadruplex structure by monitoring the inter-quartet distances (Fig. 6c, d ). The stacking pattern remained intact, for K + -stabilized MG / h-TELO , as evident from comparable distance distribution. In contrast, the stacking interactions were perturbed for MG / h-TELO in Na + media.The distance between Tetrad 1 and Tetrad 2 increases and the distance between Tetrad 2 and Tetrad 3 is widely distributed, indicating structural changes in the quadruplex topology in Na + media. CD spectroscopy also indicates that G-quadruplex exist in different conformations in the presence of other alkali metal ions than in K + (Supplementary Fig. 25 ). Therefore, MG / h-TELO may regulate ion transport by changing its conformation in response to different ions. The simulation data further complemented the results of the melting study which indicated that the stability of the MG / h-TELO is maximum in K + media (Fig. 1d ). The measurement of reversal potentials was also performed to investigate the relative permeability of different ions in comparison with K + through MG/ h-TELO ionophore. To stabilize the ionophores, it is important to use K + containing buffer in the cis side of the NPC chip (external side, i.e., the side of the addition of MG/ h-TELO ). We used a bi-ionic system of 10 mM HEPES buffer containing 0.15 M KCl in the cis side and 0.15 M different metal chlorides (internal side, i.e., LiCl, NaCl, KCl, RbCl, and CsCl) in the trans -side [59] . The holding potential was first increased to +100 mV and then switched to various testing potentials (−90 mV to +70 mV). The reversal potential was measured from an I – V curve, constructed from tail currents recorded at each potential (Supplementary Fig. 26 ). Under these conditions, control vesicles exhibited no change in current at different voltages. Upon addition of 60 μM MG/ h-TELO , different current (I) values corresponding to different voltages were recorded. The reversal potential value for 0.15 M KCl in the trans side showed value close to 0 mV, indicating that MG/ h-TELO exhibits almost equal permeability of ions (Fig. 6e, f ). On the other hand, reversal potentials of +11 mV for NaCl (permeability ratio P K + / P Na + = 2.1) and +30 mV to +67 mV were observed for 0.15 M LiCl, RbCl, and CsCl, respectively, yielding a permeability ratio ( P K + / P M + ) in the range of 3.8–7.9. These results strongly suggest that MG/h-TELO ionophore preferentially transports  K + ions. Inhibition and switching activity of the ionophore Since the binding of MG with h-TELO is pivotal for the formation of ionophore, the ion transportation can be inhibited by (i) the displacement of MG from h-TELO by a high affinity ligand like thiazole orange (TO) and (ii) disruption of MG and h-TELO interaction by cytosine. Upon addition of TO (60 μM), a complete disappearance of the transport activity of MG /h-TELO ionophore across the lipid bilaye was observed (Fig. 7a ). As TO binds to h-TELO with higher affinity compared with MG ( K D (TO) = 0.5 μM vs. K D ( MG ) = 3.2 μM), it could displace MG from h-TELO and disrupt membrane transport by the ionophore. Fig. 7: Inhibition of ion transport. Single-channel current traces recorded in the presence of MG / h-TELO (60 μM) in 1 M symmetrical KCl solution at +30 mV ( a ) showing the disappearance of ion-transport activity upon treatment with thiazole orange (TO) (4 equiv. of MG ) (pink arrow) and b inhibition in ion-transport activity upon addition of cytosine (3 equiv. of MG ) and the reversal of ion-transport activity for three cycles with addition of MG / h-TELO (2 equiv. MG over cytosine in each cycle, cyan arrow). CD spectra of MG / h-TELO in vesicles in 10 mM HEPES buffer containing 1 M KCl (pH 7.4) (purple) and the CD spectra of initial supernatant after separating vesicles by centrifugation (black line). Gradual increase in CD intensity upon addition of c TO (0–4 equiv. of MG ) and d cytosine (0–3 equiv. of MG ). Source data are provided as a Source Data file. Data are means ± SD ( n = 3). Full size image A sharp decrease in conductance was also observed when 3 equiv. excess of cytosine was added to the MG / h-TELO in the lipid bilayer (Fig. 7b ). Interestingly, the ionophoric activity could be triggered again by addition MG / h-TELO (2 equiv. excess of cytosine added). However, the conductance values were slightly decreased with each cycle and completely reduced after three cycles. The release of h-TELO from the ionophore in the lipid bilayer by TO and cytosine was monitored by CD spectroscopy (Fig. 7c, d ). The CD spectra of MG / h-TELO containing vesicles in K + buffer showed a positive peak at 290 nm and a shoulder at 270 nm. By separating the MG / h-TELO containing vesicles by centrifugation, no detectable amount of h-TELO in the supernatant was observed. However, the addition of aliquots of TO or cytosine to the mixture resulted in a gradual increase in the amount of h-TELO in the supernatant as evidenced by the appearance of the characteristic peaks for the h-TELO . These results suggest that TO and cytosine can disrupt the structure of the MG / h-TELO ionophore in the membrane. Ion-transport across the cell membrane by the MG/ h-TELO Voltage clamp measurements were performed to demonstrate the ability of the ionophore to transport K + ions across the membranes of Chinese hamster ovary (CHO) and human erythroleukemia (K-562) cell lines (10 mM HEPES, 150 mM KCl, pH 7.4) (Fig. 8a–c ; Supplementary Fig. 27 ). The control experiments revealed that CHO cells did not exhibit any endogenous ionophoric activity and K-562 cells showed weak ionophoric activity (conductance values in the range of 0.08 nS). Upon attaining the giga seal condition in both cell membranes, MG / h-TELO ionophore was added to the cis side. Under these conditions, MG / h-TELO ionophore exhibited voltage dependent K + ion conductance and two distinct open and closed states across CHO and K-562 cells. The I – V plots indicated that the ionphore shows conductance values of 1.8 nS and 2.1 nS in CHO and K-562 cell membranes, respectively (Fig. 8d, e ). These experiments demonstrate that the h-TELO ionophore can transport K + across the cell membrane. Fig. 8: Ion conductance studies across cell membrane by MG/ h-TELO . Single-channel current traces recorded at −60 mV (CHO cells) ( a ), +50 mV (CHO cells) ( b ), and +50 mV (K-562 cells) ( c ) in holding potentials in symmetrical solution of 10 mM HEPES, 150 mM KCl, pH 7.4 in the presence of MG / h-TELO (60 μM). All point histograms generated from the corresponding current traces at +50 mV and −60 mV have been presented on the right. c I − V plot using a voltage ramp (−60 mV to +60 mV) in 10 mM HEPES, 150 mM KCl, pH 7.4 symmetrical buffer in the presence of MG / h-TELO (60 μM) in CHO cells ( d ) and in K-562 cells ( e ). The red line in e shows the transport in control K-562 cells. Source data are provided as a Source Data file. Data are means ± SD ( n = 20). Full size image In this work, an ionophore is constructed from lipophilic guanosine derivative ( MG ) and h-TELO G-quadruplex. The resulting quadruplex DNA ionophore transports K + -ions across the biological membranes (Supplementary Movie 1 ). FRET melting, fluorescence titration, and ITC experiments establish that MG binds to h-TELO with a 3:1 stoichiometry. MD simulation studies reveal that the lipophilic chains of MG anchors the h-TELO and stabilizes  it within the lipid bilayer to form the ionophore. Fluorescence-based vesicle assays, voltage clamp, and MD simulation experiments collectively suggest that MG /h-TELO ionophore preferentially transports K + ions over other alkali cations. The ionophore presumably transports ions by changing its conformation in response to different ions. The reversal potential experiments suggested that the ionophore has relative permeability for K + ions over different cations in the order P K + > P Na + > P Rb + > P Li + > P Cs + (1.0:2.1:3.8:5.7:7.9). The ion transport can be disrupted by the addition of thiazole orange or cytosine. Interestingly, by carefully regulating the addition of MG / h-TELO and cytosine, a switch ON/OFF activity of the ionophore up to three cycles is achieved. Voltage clamp experiments demonstrate h-TELO ionophore transports K + ions across CHO and K-562 cell membranes. Taken together, simple and viable strategy is presented to device selective DNA based ionophores, which may provide opportunities for specific targeting of cellular receptors. Furthermore, the mechanistic details of G-quadruplex-based ionophores would provide insight into controlled ion transport for biomedical applications. General information The general chemicals and DNA sequences required for biophysical analysis were purchased from Sigma-Aldrich and IDT (USA), respectively. The DNA sequences of highest purity were purchased for best results. The lipid and cholesterol were purchased from Sigma-Aldrich. The voltage clamp studies were performed using Nanion port-a-patch (Germany) system. The details for synthetic materials and procedures have been described in Supplementary Information . LUV preparation for HPTS experiments Large unilamellar vesicles (LUVs) were formed using a 20 µL 9:1 mixture of 10 mM DphPC (1,2-diphytanoyl-sn-glycero-3-phosphocholine) and cholesterol in chloroform. After solvent removal and vacuum drying, the resulting thin film was hydrated with 500 µL of buffer (10 mM HEPES, 100 mM NaCl or KCl, pH 6.4) containing 10 µM HPTS (8-hydroxypyrene-1,3,6-trisulfonic acid trisodium salt). Next, the suspension was subjected to six freeze–thaw cycles (liquid nitrogen/water at room temperature) during hydration. The resulting white suspension was then extruded 19 times through a 100 nm polycarbonate membrane to obtain large unilamellar vesicles (LUVs) with an average diameter of ~100 nm. The LUVs suspension was separated from extravesicular HPTS dye by using size-exclusion chromatography (Econo-Pac 10DG column, Bio-rad; mobile phase: 10 mM HEPES, 100 mM NaCl or KCl, pH 6.4) and diluted with mobile phase to desired working concentration. Cation transport experiments In a clean and dry fluorescence cuvette, 5 µL of stock HPTS containing vesicle solution was suspended in 495 µL of the corresponding buffer (10 mM HEPES, 100 mM KCl, NaCl, LiCl, NH 4 Cl, and CsCl pH 6.4). Rb salts somehow interfered with the assay and hence excluded. The fluorescence of HPTS at 510 nm was monitored upon excitation at 460 nm in a time-dependent manner. For pH gradient-mediated transport experiments, different concentrations of MG/ h-TELO (0, 10, 20, 30, 40, 50, 60 μM) were mixed initially (at t = 0 s) with vesicles. At t = 50 s, 7.25 µL of aqueous NaOH (0.5 M) was added, resulting in a pH increase by one unit in the extravesicular solution. Finally, at 350 s, the vesicles were lysed with detergent (10 µL of 5% aqueous Triton X-100) resulting in the destruction of pH gradient. Molecular dynamics simulations All the simulations were performed using GROMACS 2016 molecular dynamics package [55] , [56] . A modified force field particularly developed for DNA simulation, parmbsc1 [54] , and SPC/E [60] water model was used throughout the study. Details of the system preparation, validation for the force field, and simulation methodology are provided in Supplementary Information (Molecular modeling studies, Supplementary Information). Previously, ion-channel formation by porphyrin-tagged duplex DNA was studied using atomistic simulations [31] . Motivated from the simulation protocol; here we have studied the detailed mechanism of ion-channel formation by non-covalent MG/ h-TELO assembly. Briefly, parallel G-quadruplex structure of the human telomeric DNA ( h-TELO ) was obtained from the Protein Data Bank (PDB ID: 1KF1). All-atom structure of the lipid bilayer structure was obtained from the Lipidbook [61] . Slipid force field [62] for the lipid bilayer was imported within the parmbsc1 force field and used for the simulation. Ligand ( MG ) parameters for the parambsc1 were generated using Antechamber tools [63] and Antechamber Python Parser interface (ACPYPE) [64] . MG/ h-TELO assemblies with 1:1, 2:1, and 3:1 were obtained from stepwise docking procedure using AutoDock 4.2. Each assembly was initially minimized in vacuo and then immersed into a cubic box containing SPC/E water. Appropriate numbers of K + ions were added to make each system charge neutral. All the systems were energy minimized in water using steepest descent algorithm, followed by 1 ns position restrained simulation in NPT ensemble. Finally, 500 ns of production simulations were performed in NPT ensemble at 298 K by employing Berendsen thermostat, and pressure was kept constant by coupling with Berendsen barostat. Electrostatic interactions were computed using the Particle Mesh Ewald (PME) summation method. Then a systematic procedure was followed to construct the membrane-spanning ionophore. The equilibrated bilayer was then replicated to generate a bilayer of 512 lipids. The bilayer was then solvated and subjected to 200 ns equilibrium run in NPT ensemble at 298 K. The 3:1 MG / h-TELO assembly was inserted within the large hydrated bilayer in such a way that K + -filled pores of the h-TELO were aligned along the Z -axis. The system was then subjected to 1 ns membrane insertion simulation using the membed protocol at 298 K. The system was then made charge neutral by adding appropriate number of K + and Cl − ions, such that the final salt concentration of the system became 200 mM. The system was then energy minimized, followed by 100 ns position restrained simulation in NPT ensemble at 298 K. Finally, 200 ns production run was performed in NPT ensemble. An additional system was constructed: MG / h-TELO containing Na + ions and the bulk solution containing equivalent concentration of NaCl. 100 ns position restrained simulation in NPT ensemble at 298 K was performed for each system. Finally, 200 ns production run was performed in NPT ensemble for each system. To measure the ionic current conducted by the ionophore computationally, simulations were carried out in NP z AT ensemble in presence of an external applied electric field (Supplementary Notes in Supplementary Information). Briefly, a voltage drop across the system was generated by applying an external electric field along the Z -axis. Nosé-Hoover thermostat was used to maintain temperature of the simulation at 298 K with a time constant of 0.2 ps for coupling. Area of the X–Y plane remains constant throughout the simulation timescale. Semi-isotropic pressure coupling was applied along the Z -axis using Berendsen barostat with a time constant for coupling set to 5 ps and a compressibility of 4.5 × 10 −5 bar −1 along the Z -axis. External electric field with appropriate strength was applied along the Z -axis, such that the specific voltage drop was attained. We have used the total intensity method [57] , [58] to compute the instantaneous current conducted by each system in presence of a voltage gradient across the system. Preparation of giant unilamellar vesicles (GUVs) GUVs were prepared by electroformation technique (Vesi Prep Pro, Nanion, Germany). In total, 10 µL of a 10 mM solution of DphPC and cholesterol (9:1) in chloroform was spread evenly on the indium tin oxide (ITO)-coated glass slides within the “O” ring area. The solvent was evaporated at room temperature, and the slides were dried overnight under vacuum. Then, ITO slides were assembled in the Vesi Prep Pro and filled with 275 µL of sorbitol solution (1 M). A sinusoidal AC field of 3 V and 5 Hz was applied for 2 h at 25 °C temperature. The GUV solution prepared was collected and stored at 4 °C. 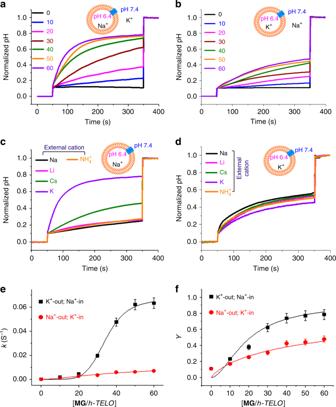Fig. 2: Fluorescence-based ion-transport assay. Change in normalized pH inside LUV (pHin) as a function of time with increasing addition ofMG/h-TELO(0–60 μM) in the presence of different metal ions and pH gradient.aBuffer composition, external: 10 mM HEPES, 100 mM KCl, pH 7.4; internal: 10 mM HEPES, 100 mM NaCl, pH 6.4.bBuffer composition, external: 10 mM HEPES, 100 mM NaCl, pH 7.4; internal: 10 mM HEPES, 100 mM KCl, pH 6.4. Change in normalized pH inside LUV as a function of time in the presence ofMG/h-TELO(60 μM) using different external metal ions.cBuffer composition, external: 10 mM HEPES, 100 mM MCl (M = Na+, Li+, Cs+, NH4+, and K+), pH 7.4; internal: 10 mM HEPES, 100 mM NaCl, pH 6.4.dBuffer composition, external: 10 mM HEPES, 100 mM MCl (M = Na+, Li+, Cs+, NH4+, and K+), pH 7.4; internal: 10 mM HEPES, 100 mM KCl, pH 6.4.ePseudo-first-order initial constant rate as a function of final concentration ofMG/h-TELOin the bilayer membrane.fFractional activity Y = f([MG/h-TELO]) plotted for Na+and K+ions and the curves are the best fit from the Hill equation. Source data are provided as a Source Data file. Data are means ± SD (n= 3). Conductance measurements in vesicles Conductance measurements were performed using the Port-a-Patch setup (Nanion, Munich, Germany). First, a borosilicate glass chip (NPC chip, Nanion, Germany) with 3–5 mΩ was loaded with symmetrical working buffers containing 1 M MCl (M = Li + , Na + , K + , Rb + , NH 4 + , Li + , and Cs + ), and 10 mM HEPES (pH 7.0) in both cis and trans compartments and Ag/AgCl electrodes were placed on both sides of the NPC chip. Next, bilayer membrane with >1 Giga Ohm resistance was constructed across the micrometer-sized aperture in the NPC chip by adding GUV suspension and applying a small negative pressure (−20 mbar). MG/ h-TELO (60 μM) was added to the cis side of the chamber. Current traces were recorded using an HEKA EPC 10 patch clamp amplifier with a built-in 1 kHz 4 pole Bessel low-pass filter and a Digidata 1322 A digitizer. The I–V curve was generated using a voltage ramp from −60 mV to +60 mV. For ion-transport inhibition, TO (4 equiv.) and cytosine (3 equiv. of total MG concentration) to the cis side after a stable ion transport by MG/ h-TELO was established. Data analysis was performed using Clampfit 10.6 software. Cell culture and voltage–clamp measurements in cells CHO (ATCC) and K-562 (National Centre for Cell Science (NCCS), Pune, India) cells were cultured in 25 cm 2 flasks in DMEM (high glucose) and 1:1 F12K/DMEM supplemented with 10% FBS (GIBCO, heat inactivated, US origin, catalogue number 10082147) at 37 °C, 5% CO 2 . Cells were harvested, and the culture media was substituted with external solution (10 mM HEPES, pH 7.4) with 150 mM of KCl. For these experiments, we have used 3–5 mΩ NPC chips to form bilayer across its micrometer-sized aperture. Next similar to vesicle experiments, the MG/ h-TELO (60 μM) was added to the cis side of the chip, and the data were recorded. For each type of cells, we performed 20 replica experiments and analyzed the data. The data acquisition and analysis were carried out similar to vesicle experiments. 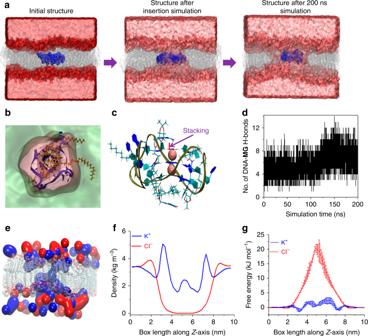Fig. 3: MG/h-TELOionophore formation within lipid bilayer. aProcess of pore formation aroundh-TELOwithin the lipid membrane. Initially, ligand-bound quadruplex (blue vdW representation) is placed within the lipid bilayer (gray stick) in a water box (red surface).bFinal structure of the supramolecular quadruplex-based ion pore. Lipid bilayer is colored in green surface, whereas the water pore surrounding the quadruplex is shown in pink surface.h-TELOis shown in blue cartoon, and boundMGis shown in orange sticks.cStructure ofMG/h-TELOis shown. G-quadruplex is shown in cartoon representation, whereas bound ligand is shown in stick mode.dThe number of hydrogen bonds betweenh-TELOandMGduring the simulation of the ionophore is shown.eA representative snapshot of K+(blue) and Cl−(red) ion distributions in the simulation box is shown. Lipid bilayer is shown as gray transparent surface.fDensity profiles of K+(blue) and Cl-(red) ions averaged over the entire 200 ns simulation trajectory are shown.gPotential of mean force profile for K+(blue) and Cl−(red) translocation across the simulation box (Z-axis). Source data are provided as a Source Data file. Data are means ± SD (n= 3). Statistics Results are expressed as means ± SD of n number of independent experiments. 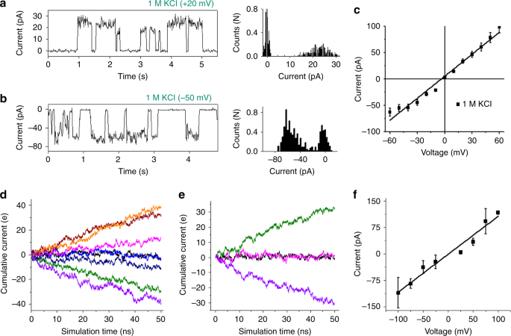Fig. 4: Ion conductance studies across the lipid bilayer by MG/h-TELO. Single-channel current traces recorded at +20 mV (a) and −50 mV (b) holding potentials in 1 M symmetrical KCl solution in the presence ofMG/h-TELO(60 μM). All point histograms generated from the corresponding current traces at +20 mV and −50 mV have been presented on the right.cI−Vplot using a voltage ramp (−60 mV to +60 mV) in 1 M symmetrical KCl solution (black line) in the presence ofMG/h-TELO(60 μM). Data are means ± SD (n= 3).dCumulative currents through the transmembrane pore resulting from the application of external electric fields. Orange, maroon, pink, black, light blue, deep blue, green, and purple color represent +100 mV, +75 mV, +50 mV, +25 mV, −25 mV, −50 mV, −75 mV, and −100 mV applied voltage biases.eCumulative current flow for K+ions under the applied voltage biases of +100 mV (green), −100 mV (purple) and for Cl−ions under the applied voltage biases of +100 mV (black), −100 mV (pink).fCurrent/voltage characteristics of supramolecular transmembrane ionophore computed from molecular dynamics simulations under different applied voltage biases. Source data are provided as a Source Data file. Data represented as Mean ± SD (n= 4). 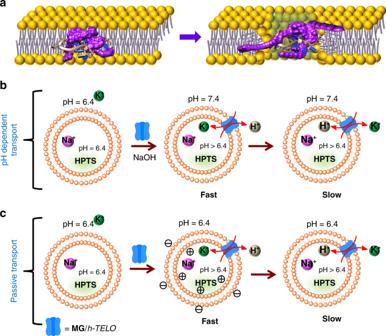Fig. 5: Proposed mechanism for ion transport in fluorescence assay. Schematic representation showingathe formation of water-filled ionophore in the lipid bilayer by rearrangement of lipid molecules upon insertion ofMG/h-TELO. The lipophilic chains ofMGanchors theMG/h-TELOto stabilize the ionophore.bThe stepwise ion transport (left to right) by pH-dependent transport (top) and;cpassive diffusion (bottom). 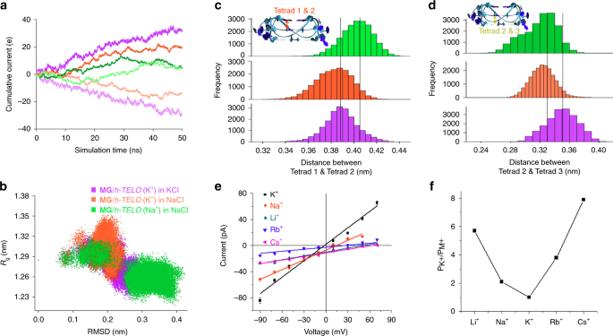Fig. 6: MG/h-TELOas K+ionophore. Molecular dynamics simulations ofMG/h-TELOin KCl and NaCl electrolyte solutions, represented by purple and orange color, respectively. The Na+-stabilizedMG/h-TELOin NaCl electrolyte solution is represented by green color.aCumulative current flow computed for the three systems under the applied voltage biases of +75 mV, rendered in the dark color and −75 mV, represented in light color.b2-D scatter plot of root-mean-square deviation (RMSD) and radius of gyration (Rg) obtained from the equilibrium simulations. Variations of the distance vector along theZ-axis between tetrads 1 & 2cand tetrads 2 & 3dare shown forMG/h-TELOionophore embedded in the lipid bilayer in three different conditions obtained from the simulations.eI–V curves generated from the tail currents of the traces in different buffer conditions. Bi-ionic conditions were used: 10 mM HEPES buffer containing 0.150 M KCl in thecisside and 0.150 M different metal chlorides (LiCl, NaCl, KCl, RbCl, and CsCl) in thetransside.fPermeability ratios ofMG/h-TELOobtained for different monovalent cations with respect to K+ion. Source data are provided as a Source Data file. Data represented as mean ± SD (n= 4). 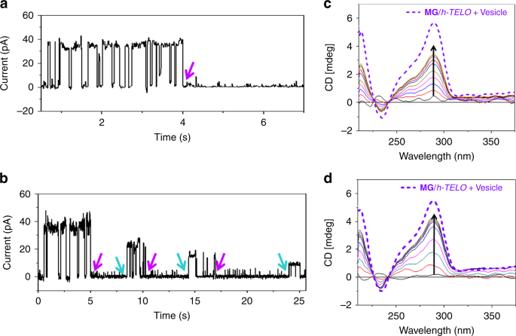Fig. 7: Inhibition of ion transport. Single-channel current traces recorded in the presence ofMG/h-TELO(60 μM) in 1 M symmetrical KCl solution at +30 mV (a) showing the disappearance of ion-transport activity upon treatment with thiazole orange (TO) (4 equiv. ofMG) (pink arrow) andbinhibition in ion-transport activity upon addition of cytosine (3 equiv. ofMG) and the reversal of ion-transport activity for three cycles with addition ofMG/h-TELO(2 equiv.MGover cytosine in each cycle, cyan arrow). CD spectra ofMG/h-TELOin vesicles in 10 mM HEPES buffer containing 1 M KCl (pH 7.4) (purple) and the CD spectra of initial supernatant after separating vesicles by centrifugation (black line). Gradual increase in CD intensity upon addition ofcTO (0–4 equiv. ofMG) anddcytosine (0–3 equiv. ofMG). Source data are provided as a Source Data file. Data are means ± SD (n= 3). 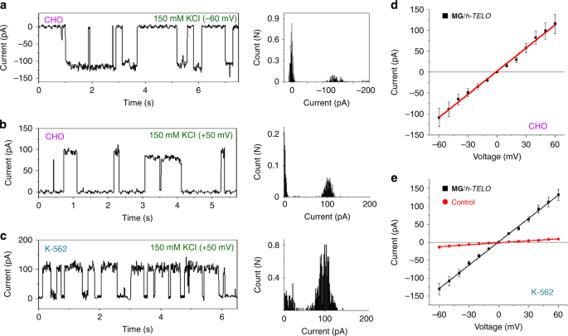Fig. 8: Ion conductance studies across cell membrane by MG/h-TELO. Single-channel current traces recorded at −60 mV (CHO cells) (a), +50 mV (CHO cells) (b), and +50 mV (K-562 cells) (c) in holding potentials in symmetrical solution of 10 mM HEPES, 150 mM KCl, pH 7.4 in the presence ofMG/h-TELO(60 μM). All point histograms generated from the corresponding current traces at +50 mV and −60 mV have been presented on the right.cI−Vplot using a voltage ramp (−60 mV to +60 mV) in 10 mM HEPES, 150 mM KCl, pH 7.4 symmetrical buffer in the presence ofMG/h-TELO(60 μM) in CHO cells (d) and in K-562 cells (e). The red line ineshows the transport in control K-562 cells. Source data are provided as a Source Data file. Data are means ± SD (n= 20). Reporting summary Further information on research design is available in the Nature Research Reporting Summary linked to this Article.